Reply to: The pitfalls of interpreting hyperintense FLAIR signal as lymph outside the human brain 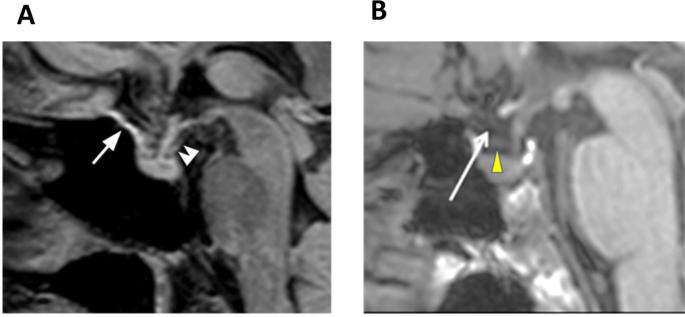Fig. 1: Visualization of the diaphragma sella. ASagittal FLAIR images show the putative ventral dural lymphatic elements in the diaphragma sella (double arrowhead; (adapted from Figure 4c of Albayram et al.,Nat. Commun. 13, 203 (2022)1).BMoreover, we can identify a subtle linear pattern, most likely the diaphragma sella (yellow arrowhead) in Ringstad et al. Figure 1c2, just under their arrow, as presented below (with contrast adjustment); (adapted from Fig. 1c at Rinstad et al.,Nat. Commun. submitted). Further information on research design is available in the Nature Portfolio Reporting Summary linked to this article.